Cell dipole behaviour revealed by ECM sub-cellular geometry Cells sense and respond to their mechanical environment by exerting forces on their surroundings. The way forces are modulated by extra-cellular matrix (ECM) properties plays a key role in tissue homoeostasis. Using highly resolved micropatterns that constrain cells into the same square envelope but vary the adhesive geometry, here we investigate how the adhesive micro-environment affects the architecture of actin cytoskeleton and the orientation of traction forces. Our data demonstrate that local adhesive changes can trigger orientational ordering of stress fibres throughout the cell, suggesting that cells are capable of integrating information on ECM geometry at the whole-cell level. Finally, we show that cells tend to generate highly polarized force pattern, that is, unidirectional pinching, in response to adequate adhesive conditions. Hence, the geometry of adhesive environment can induce cellular orientation, a process which may have significant implications for the formation and mechanical properties of tissues. Within living tissue, cells are able to gather information from their environment by exerting forces on the extra-cellular matrix (ECM), a process which is essential for the maintenance of cell shape and function. Many studies have pointed out that the physical properties of the ECM, such as geometry [1] rigidity [2] , [3] and topography [4] , [5] , can influence the forces exerted by cells which in turn affect cell shape and ultimately lead to the modification of crucial cellular processes, ranging from migration to differentiation [6] , [7] , [8] . However the interplay between ECM properties and cell cytoskeletal architecture and the related tensional forces are far from being completely understood. To build a complete picture, one would need to determine the cellular response to each specific cue from the environment. Such measurement would be difficult in in vivo environments, in which complexity induces a large variability in cell behaviour. One strategy is to place cells in a normalized, reproducible environment where it is straightforward to measure the influence of a given parameter. For this reason, microfabrication techniques [9] , [10] , [11] , [12] , [13] have been used to produce patterns of adhesive proteins, which made it possible to study cells with a well-defined shape. Cell shape was shown to play a role in various cellular processes, such as focal adhesion (FA) assembly [14] or stem cell lineage commitment [15] . More recently, micropatterning on soft substrates [16] , [17] has allowed the measurement of traction forces associated with a given cell shape. In this way, traction forces were found to increase with the cell spreading area [18] , [19] . Cell aspect ratio was also shown to have a strong impact on cellular force distribution [20] , [21] , as well as the differentiation of mesenchymal stem cells [8] . In these studies on soft substrates, adhesive patterns with convex shapes, such as filled disks [16] , squares or rectangles [8] , [21] , have been used. Such patterns make it possible to control the overall shape and area of cell envelope but do not allow to modulate the internal cytoskeletal organization independently from the cell envelope. In this study, we investigate the influence of sub-cellular adhesive geometry on cytoskeleton organization and traction forces, using highly resolved soft substrate micropatterns that make it possible to define the adhesive geometry at the sub-cellular level while keeping the overall cell envelope unchanged. To control cells internal cytoskeletal organization, we fabricated soft substrate micropatterns with high spatial resolution to define the adhesive geometry at the sub-cellular level while keeping the overall cell envelope unchanged. The patterns were designed to confine the cell in a square envelope, that would remain virtually unaffected, while varying the adhesive properties on the sides of the square. It has been shown, for micropatterns on glass substrates [1] that actin bundles form predominantly over non-adhesive borders. Therefore, we chose to vary the number and position of non-adhesive edges, and study the response of the cell in terms of cytoskeleton architecture and cell-generated forces. We believe that this approach would allow us to untangle the effect of cell shape/area from that of sub-cellular cell organization on traction forces, using a reductionist system based on micropatterns. In the following, while similar cell envelopes are maintained, we present the impact of sub-cellular adhesive geometry on the spatial organization of actin and FAs, the total cell contractility and the localization of traction stress. Force dipole analysis is used to determine the principal orientation and the degree of cell polarization. Traction force orientation is correlated with the directions of actin stress fibres. We show that cells integrate information on ECM geometry at the whole-cell level. Specific sub-cellular ECM geometry can trigger a reorganization of the actin cytoskeleton and induce cell polarization, while the cell shape remains unchanged. Pattern geometry and resulting cytoskeletal organization Since our aim is to study cells with an identical shape, cell spreading is controlled using square adhesive islands of 900 μm 2 projected area with 7 μm-wide adhesive bars, which are created on 5 kPa polyacrylamide (PAA) hydrogels by deep ultraviolet illumination. The engineered substrates are incubated in a solution containing a mixture of fibronectin and fluorescent fibrinogen, so that the resulting adhesive pattern can be imaged by fluorescence microscopy. To control the cytoskeletal architecture, the pattern geometry is designed to alternate between adhesive and non-adhesive regions at the cell edge. Since previous studies [1] have shown that cells tend to form reinforced actin fibre bundles along non-adhesive edges, we aimed at modulating the cytoskeletal organization by varying their number and positions. Three different micropatterns, printed on the same coverslip, were used: [U], [H] and [ARROW] ( Fig. 1 ). Within 2 h after being plated onto the substrate, a large majority of cells adopted square shapes of approximately equal projected area. 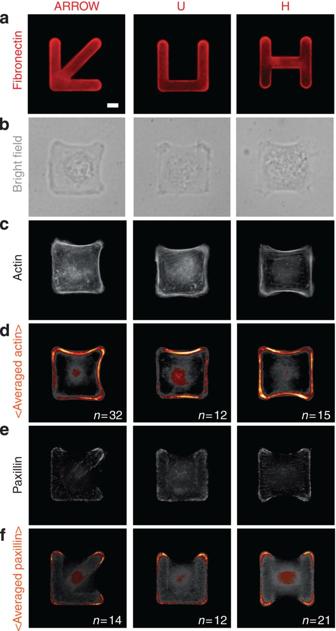Figure 1: Cell cytoskeleton responds to adhesive micropattern geometry on soft substrates. (a) [ARROW]-, [U]- and [H]-shaped fibronectin micropatterns on polyacrylamide hydrogels. The chosen patterns [U], [H] and [ARROW] present, respectively, one, two independent and two connected non-adhesive edges. Each pattern envelope corresponds to an equivalent projected area of 900 μm2. (b) Bright-field images show that MEF cells follow similar square shapes on all three patterns. (c) Individual actin-labelled cells. (d) Average actin image overncells. Actin is localized preferentially along the cell periphery, with fibres present along adhesive and non-adhesive edges. (e) Individual cell with paxillin staining, revealing focal adhesion localization. (f) Average paxillin images show that focal adhesions are located on the outer edge of the adhesive patterns and more concentrated at cell apices in correlation with stress fibre ends. (Scale bar, 7 μm). Figure 1: Cell cytoskeleton responds to adhesive micropattern geometry on soft substrates. ( a ) [ARROW]-, [U]- and [H]-shaped fibronectin micropatterns on polyacrylamide hydrogels. The chosen patterns [U], [H] and [ARROW] present, respectively, one, two independent and two connected non-adhesive edges. Each pattern envelope corresponds to an equivalent projected area of 900 μm 2 . ( b ) Bright-field images show that MEF cells follow similar square shapes on all three patterns. ( c ) Individual actin-labelled cells. ( d ) Average actin image over n cells. Actin is localized preferentially along the cell periphery, with fibres present along adhesive and non-adhesive edges. ( e ) Individual cell with paxillin staining, revealing focal adhesion localization. ( f ) Average paxillin images show that focal adhesions are located on the outer edge of the adhesive patterns and more concentrated at cell apices in correlation with stress fibre ends. (Scale bar, 7 μm). Full size image First, we examined actin cytoskeletal architecture and FA formation on these micropatterns. To do this, samples were fixed, immunofluorescently probed for F-actin and paxillin and imaged using epifluorescence microscopy. The resulting images are shown in Fig. 1 for single cells as well as the images obtained by averaging over many cells that provide a population insight. Actin fluorescence images show that actin is localized preferentially along the cell periphery. However, contrary to observations on glass substrate [1] , averaged cells do not show a significant reinforcement of actin along non-adhesive edges. Stress fibres are present along the four sides of the square envelope, and non-supported fibres (NSF) are not characterized by a visible actin enrichment. Similar observations have been reported, showing that reinforced NSFs appear when the local stiffness increases [22] . Paxillin images, which reveal the localization of FA, have also been recorded for many cells and averaged ( Fig. 1e,f ). FAs appear most prominent on the outer edge of the adhesive patterns corresponding to the cell borders. A higher concentration is observed at cell apices in good correlation with the localization of actin fibre ends. On [U] shape, paxillin maps show a slight enrichment of FAs in the upper corners adjacent to the non-adhesive edge. The paxillin localization observed on the [ARROW] shape also confirms this effect: FA is enhanced in the upper-right corner, corresponding to the ends of two NSFs. Since it is known that tensional forces transmitted through integrin receptors can modulate FA assembly [23] , [24] , [25] , this local enrichment in FA is an indication that NSF exert more tension than SF formed along adhesive regions. Total contractile energy and stress localization For traction force measurements, Mouse Embryonic Fibroblasts (MEFs) (kindly provided by Corinne Albigès-Rizo’s lab) were plated on the micropatterns and used for patterned traction cytometry. Spread cells exerted traction forces on the substrate that induced the displacement of fluorescent nanobeads embedded in the gel. Traction forces were calculated, using Fast Fourier Transform Traction Cytometry [26] , [27] , from measured beads displacements which were obtained by a combination of particle imaging velocimetry and single particle tracking, as described previously [28] . Throughout the experiments, gel stiffness was kept constant at 5 kPa and, to obtain comparable measurements, the cells were cultured on a single coverslip where micropatterns of all shapes were present. First we studied the overall contractility level. Previous studies have suggested that actin reinforcement triggers the activation of a positive feedback loop [29] , [30] between tension in the actin cables and FA maturation that ultimately leads to a local increase of traction forces. To examine whether the presence of NSF would impact the magnitude of traction forces at the cell level, [U] and [H] shapes are designed to induce either one or two NSF of equal length on cells of identical envelope, while [ARROW] shape produces two NSFs with a common anchor to concentrate local strain which may, through a feedback mechanism, lead to an increase of traction force. We calculated the total contractile energy generated by cells on the three patterns, which is obtained by integrating the scalar product of the stress and displacement vectors across the entire cell surface. Interestingly, there is no significant difference in the level of contractility between the three shapes [U], [H] and [ARROW] ( Fig. 2a ). This lack of difference between the three patterns suggests that, for a given envelope, cells tend to maintain a fixed amount of tension, regardless of the ECM geometry. 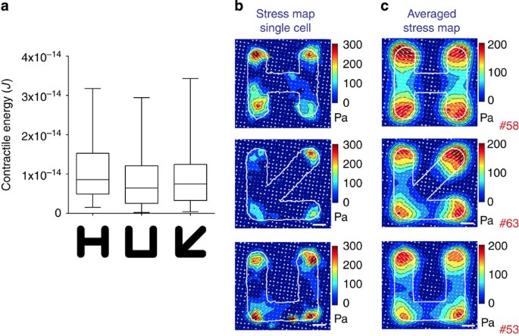Figure 2: Cells of similar shape maintain a fixed amount of contractile energy regardless of the adhesive geometry. (a) Contractile energy of cells of similar envelope plated on [ARROW] (n=63), [U] (n=53) and [H] (n=58) soft micropatterns. Error bars represent s.e.m. Using one-way analysis of variance with the Tukey’s honestly significant differencepost-hoctest, no significant differences are found between the contractility of cells on the three micropatterns (b) Individual stress maps calculated by Fourier Transform Traction Cytometry show that traction forces tend to be localized at cell corners, in spite of the inter-cellular variability. (c) Averaged stress maps obtained from ~50 cells per shape confirm that forces are mainly localized at the corners of the square envelope, with enhanced traction stress at corners adjacent to a non-adhesive edge. (traction magnitude is given in Pascals.). Figure 2: Cells of similar shape maintain a fixed amount of contractile energy regardless of the adhesive geometry. ( a ) Contractile energy of cells of similar envelope plated on [ARROW] ( n =63), [U] ( n =53) and [H] ( n =58) soft micropatterns. Error bars represent s.e.m. Using one-way analysis of variance with the Tukey’s honestly significant difference post-hoc test, no significant differences are found between the contractility of cells on the three micropatterns ( b ) Individual stress maps calculated by Fourier Transform Traction Cytometry show that traction forces tend to be localized at cell corners, in spite of the inter-cellular variability. ( c ) Averaged stress maps obtained from ~50 cells per shape confirm that forces are mainly localized at the corners of the square envelope, with enhanced traction stress at corners adjacent to a non-adhesive edge. (traction magnitude is given in Pascals.). Full size image To investigate how the spatial distribution of forces responds to ECM geometry, traction stress maps are calculated, such as the ones shown in Fig. 2b for individual cells. Because stress distribution is highly variable from cell–to-cell, an important advantage of micro-patterned experiments is the possibility to average traction force distribution from individual cells to obtain a statistically relevant force distribution [28] . We used the pattern fluorescence image as a reference to superimpose individual traction maps and calculate averaged stress maps, which are shown in Fig. 2c from more than 50 cells per shape. Traction stress appears to be localized at cell apices without major differences between adhesive and non-adhesive borders. Cells are known to present enhanced traction stress at the corners of their square envelope [12] , [16] , [21] or at apices [28] . Therefore, our results suggest that the shape of the cell envelope is the dominant factor in the distribution of traction stress. The impact of actin reinforcement along non-adhesive edge is however visible: on [U] shape, the upper corners (on both sides of the NSF) exhibit stresses that are spread over a larger area, corresponding to a superior level of force in this region, compared with the bottom corners; on [ARROW] shape, a higher level of stress can be seen at the corner where the two NSFs are focused. Detailed quantification of the forces at the four corners as a function of pattern geometry is presented in Supplementary Note 1 . Supplementary Fig. 1 shows that force magnitude increases significantly, though moderately, in the corners where NSFs are anchored. These data confirm that, when bridging over non-adhesive regions, cells reinforce their actin architecture and the associated anchorage structures, which are transduced into a local stress increase. However, this effect only accounts for variations of <20% per NSF on average, while the dominant factor governing traction magnitude distribution is the shape of the cell envelope. Force orientation reveals ECM sensing at whole-cell level In the previous paragraph, we have compared the averaged traction stress magnitude between the three shapes. Now we turn our attention to the stress local orientation. To visualize this orientation, each position on the average stress map is assigned a colour, which depends on the angle of the local stress (in our case, the reference axis is the vertical one). As an example, the schematized cell drawn in Fig. 3a shows that vertical force vectors exerted by the cell on its substrate are conveyed in blue, whereas horizontal force vectors correspond to red colour. The brightness of this colour is modulated by the stress magnitude, so that the orientation of very small forces would not be considered. The resulting maps, shown in Fig. 3 for the three shapes, are named ‘Force Orientation Maps’ (FOMs) and provide a direct visualization of the dominant orientation of traction force at each given location on the adhesive pattern. 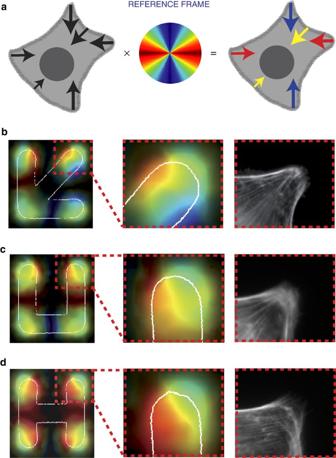Figure 3: Force Orientation Maps (FOM) reveal different actin organization in cells of similar shapes. (a) Traction stress distribution obtained from Fourier Transform Traction Cytometry were translated into FOM by assigning a colour code to each force vector depending on its orientation in a reference frame. FOM provides information locally on the orientation of the dominant stress fibres and helps visualize the contractile organization of the entire cell. (b) Average FOM for [ARROW] (n=63). The close-up on the upper-right corner displays red and blue areas related to the presence of two dominant stress direction. The image of a typical actin-stained cell in the same zone shows the corresponding fibres. (c,d) Average FOM for [U] (n=53) and [H] (n=58) with a close-up in the upper-right corner and a typical actin image of the same area. FOM of [U] and [H] are significantly different in this area while the adhesive patterns are geometrically identical: stress are mainly directed diagonally on [U] and horizontally on [H] as indicated by the red patch on the FOM. Actin images show that the stress fibres are mostly arranged horizontally in the case of [H], while they span a broad range of angles on [U]. The transition from [U] to [H] has thus induced a complete acto-myosin remodelling, suggesting that cytoskeleton organization is not only driven by local adhesive conditions but results from information on the ECM integrated at the whole-cell level. Figure 3: Force Orientation Maps (FOM) reveal different actin organization in cells of similar shapes. ( a ) Traction stress distribution obtained from Fourier Transform Traction Cytometry were translated into FOM by assigning a colour code to each force vector depending on its orientation in a reference frame. FOM provides information locally on the orientation of the dominant stress fibres and helps visualize the contractile organization of the entire cell. ( b ) Average FOM for [ARROW] ( n =63). The close-up on the upper-right corner displays red and blue areas related to the presence of two dominant stress direction. The image of a typical actin-stained cell in the same zone shows the corresponding fibres. ( c , d ) Average FOM for [U] ( n =53) and [H] ( n =58) with a close-up in the upper-right corner and a typical actin image of the same area. FOM of [U] and [H] are significantly different in this area while the adhesive patterns are geometrically identical: stress are mainly directed diagonally on [U] and horizontally on [H] as indicated by the red patch on the FOM. Actin images show that the stress fibres are mostly arranged horizontally in the case of [H], while they span a broad range of angles on [U]. The transition from [U] to [H] has thus induced a complete acto-myosin remodelling, suggesting that cytoskeleton organization is not only driven by local adhesive conditions but results from information on the ECM integrated at the whole-cell level. Full size image On the FOM displayed on Fig. 3b , the [ARROW] shape exhibits two dominant orientations (blue and red regions) at the upper-right corner, revealing the presence of the two NSFs. The most striking observation is the difference between [H] and [U] FOM around the two upper corners, in spite of the similitude between those patterns in this region. [H] micropattern FOM presents large red zones, indicating that the dominant force vector is directed horizontally, which reveals that actin fibres on [H] micropattern tend to orient perpendicularly to the two facing adhesive bars. In contrast, [U] micropattern FOM displays large green areas, indicating that forces and thus actin fibres are oriented diagonally towards the centre of the [U]. This difference suggests that a slight change in the local ECM distribution, induced by the displacement of the horizontal adhesive bar from bottom to centre, triggered a global modification of the contractile response. This seemed associated with a reorganization of the cytoskeleton, as shown by typical actin-stained cells (right-hand side of Fig. 3c,d ): actin fibres are mostly horizontal on [H], while those fibres have various directions on [U]. Actin fibre orientation are analyzed in a later section. Cell polarization can be strongly triggered by ECM geometry Since individual cell’s behaviour may be hidden in the average traction map, we performed orientation analysis at the single cell level. One way to extract the main directions from a traction map is by calculating the first order moment of the force distribution [26] , also named force dipole [31] , a 2 × 2 tensor M ij , which has the dimension of an energy and describes the contraction/dilation forces as well as the torques applied by the cell. The elements M ij are obtained by integrating the coordinate r i times the traction stress T j over the cell envelope: Since the net torque exerted by the cell is expected to be zero, the matrix M is symmetrical in theory. Hence, it is possible to find the principal contractile axes by applying a rotation operator to obtain a diagonal matrix. In this description, the force distribution is reduced to two contractile dipoles along the two principal directions. Practically, the first order moment tensor M is calculated from the experimental traction map for individual cells and the dominant orientation is determined from the direction of the eigenvector corresponding to the largest eigenvalue. This direction should indicate the cell orientation in the case of a polarized force pattern. It has been shown that, in many situations, (motile cells, strained substrate) the cell exerts an anisotropic ‘pinching’ force pattern [32] , [33] . Here we investigated if such a polarized force pattern is also found on non-migrating cells and how the dominant cell orientation is determined by the ECM geometry in the case of our three patterns. The angle of the main contraction direction relative to a reference axis (drawn in red on each shape of Fig. 4a ) is depicted as histograms on Fig. 4b . The number of cells analyzed for each micropattern is 72 for [H], 56 for [U] and 69 for [ARROW]. The most striking result is the sharp peak at 90° in the histogram of [H], corresponding to the direction perpendicular to the facing adhesive bars. A large fraction of cells (70%) have a dominant contraction oriented within 10° of this direction. [H] seems capable of inducing a preferential orientation of the force pattern in a very efficient way. In contrast, cells on [U] can adopt a wide range of orientations (from 45° to 90° relative to the symmetry axis) with equal probability. The only visible trend is their tendency to avoid the vertical direction. Concerning the [ARROW] case, cell orientations span all angles with two maxima corresponding to the direction of the diagonal bar and the orthogonal diagonal direction. One could expect that the local stress enhancement, on the upper-right corner of [ARROW], due to the junction of two NSFs would favour a force pattern along the diagonal bar. However, this effect is weak: this direction is slightly more probable but the orientation is essentially broadly distributed. 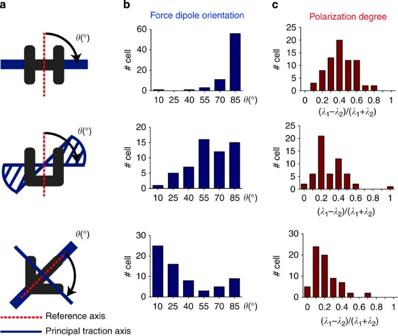Figure 4: The first moment of traction stress yields the dominant contractile orientation and the degree of polarization for each cell. (a) Micropattern drawings showing the reference axis (red line with squares) from which the angleθis defined and the most frequent directions of the principal traction (blue hatched areas) for [H], [U] and [ARROW]. (b) Direction of the principal traction calculated on individual cells ([H]:n=72, [U]:n=56 and [ARROW]:n=69). A large majority of cells are oriented within 10° of the horizontal direction on [H]. For [U] patterns, a wide range of directions from horizontal to diagonal are equally probable, while on [ARROW] contractions in the two diagonal directions are favoured. (c) The ratio (λ1−λ2)/(λ1+λ2), whereλ1andλ2are the two eigenvalues of the first moment tensor, indicates the degree of polarization of the force pattern and is found to vary significantly between the three patterns. This value is ~0.5 for [H], revealing a good degree of polarization and an unidirectional pinching force pattern. In contrast, most cells on [ARROW] exhibit a ratio closer to 0, showing a low degree of polarization. In our case, it means that all four corners of the square envelope exert similar contractions. Figure 4: The first moment of traction stress yields the dominant contractile orientation and the degree of polarization for each cell. ( a ) Micropattern drawings showing the reference axis (red line with squares) from which the angle θ is defined and the most frequent directions of the principal traction (blue hatched areas) for [H], [U] and [ARROW]. ( b ) Direction of the principal traction calculated on individual cells ([H]: n =72, [U]: n =56 and [ARROW]: n =69). A large majority of cells are oriented within 10° of the horizontal direction on [H]. For [U] patterns, a wide range of directions from horizontal to diagonal are equally probable, while on [ARROW] contractions in the two diagonal directions are favoured. ( c ) The ratio ( λ 1 − λ 2 )/( λ 1 + λ 2 ), where λ 1 and λ 2 are the two eigenvalues of the first moment tensor, indicates the degree of polarization of the force pattern and is found to vary significantly between the three patterns. This value is ~0.5 for [H], revealing a good degree of polarization and an unidirectional pinching force pattern. In contrast, most cells on [ARROW] exhibit a ratio closer to 0, showing a low degree of polarization. In our case, it means that all four corners of the square envelope exert similar contractions. Full size image The ratio r =( λ 1 − λ 2 )/( λ 1 + λ 2 ), where λ 1 and λ 2 are the two eigenvalues of the moment tensor, has a value between 0 and 1. It indicates the degree of polarity of the cell. In a purely unidirectional pinch, the eigenvalue corresponding to the principal traction would be much higher than the other one and r is close to 1, which reveals a polarized cell. On the contrary, if both directions sustain equivalent tractions, the two eigenvalues have similar magnitude and r =0. We have examined the distribution of this ratio for cells plated on the three patterns and the results are depicted on Fig. 4c . For the [ARROW] shape, cells exhibit a ratio close to 0.1, which reveals a weak degree of polarization. In contrast, the distribution of this ratio for [H] moves towards larger values, revealing a more polarized force pattern with the pinch direction orthogonal to the vertical facing bars. The eigenvalue ratio on [U] presents an intermediate degree of polarization, which is not surprising, since, in spite of the presence of two facing bars as in [H], a wide range of orientations seem to be allowed on the [U] shape. In summary, cells on [ARROW] tend to adopt a configuration with forces in the four corners directed towards the cell centre, whereas [H] seems to trigger the development of a highly polarized force pattern with predominant contraction along the horizontal bar. Finally, we have shown that ECM adhesive micro-environment can induce a global cellular response, which is evidenced by the orientation of the dominant tractions and the degree of polarization of the force pattern exerted by the cell. Actin organization is correlated with force orientation We have observed the cell response in terms of traction force orientations. Since force directions reflect the cytoskeletal architecture, our data suggests that a reorganization of the cytoskeleton is induced by ECM adhesive geometry. To confirm this assertion, we have directly studied the orientation of actin fibres in the cytoskeleton. Fixed and actin-stained cells on the three patterns have been imaged by a confocal microscope and the orientations of F-actin filaments for each cell have been analyzed using the method described in ref. 34 . For each pixel of the image, the local derivatives are computed and provide the dominant direction and degree of orientation (coherency parameter) at this location. An histogram is built from the directions, weighted by the coherency, as shown in Fig. 5d . For each cell, this angular distribution is fitted by four von Mises distributions (equivalent of Gaussian distribution in directional statistics) to yield the main orientations. Note that images of individual cells are cropped to remove the cell borders. This procedure allows to discard the impact of the bright actin fibres that are always present at the periphery and dominate the angular distribution and to focus on cytoskeleton organization specific to each pattern. To retain the principal and secondary orientation for each cell, the von Mises distributions that are too widely spread (s.d.>40°) are rejected and they are sorted in terms of their integrated surface. 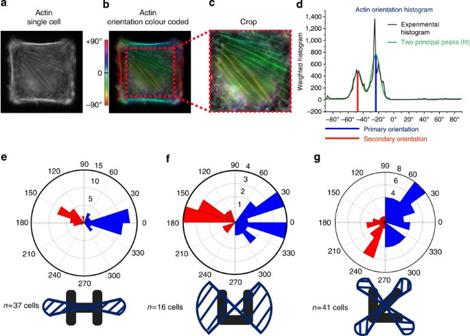Figure 5: Analysis of actin fibre orientation. (a) Individual cells on pattern imaged in confocal microscopy. (b) Colour-coded map given by OrientationJ (plugin for ImageJ) showing the angle of oriented features in the image. (c) Only the centre part of the cell is analyzed since fibres at the periphery are always at the same angle. (d) Histogram of the angle distribution in the image weighted by the coherency parameter to give more importance to pixels in locally more oriented features (black) and fit with von Mises distributions showing two principal peaks (green). The principal and second peak positions for all cells on a given pattern are shown on angle histograms (the dominant peak angle is shown in blue on the right-hand side of the plot, while the secondary peak is shown in red on the left-hand side of the plot): most angles are close to the horizontal direction on [H] patterns (e); a range of angles from ~−45° to +45° is found on [U] patterns (f); the [ARROW] pattern induced a broad angle distribution with a peak at +45° parallel to the diagonal adhesive bar (g). [H]:n=37, [U]:n=16 and [ARROW]:n=41. All angle values are relative to the horizontal of the pattern drawing. Figure 5: Analysis of actin fibre orientation. ( a ) Individual cells on pattern imaged in confocal microscopy. ( b ) Colour-coded map given by OrientationJ (plugin for ImageJ) showing the angle of oriented features in the image. ( c ) Only the centre part of the cell is analyzed since fibres at the periphery are always at the same angle. ( d ) Histogram of the angle distribution in the image weighted by the coherency parameter to give more importance to pixels in locally more oriented features (black) and fit with von Mises distributions showing two principal peaks (green). The principal and second peak positions for all cells on a given pattern are shown on angle histograms (the dominant peak angle is shown in blue on the right-hand side of the plot, while the secondary peak is shown in red on the left-hand side of the plot): most angles are close to the horizontal direction on [H] patterns ( e ); a range of angles from ~−45° to +45° is found on [U] patterns ( f ); the [ARROW] pattern induced a broad angle distribution with a peak at +45° parallel to the diagonal adhesive bar ( g ). [H]: n =37, [U]: n =16 and [ARROW]: n =41. All angle values are relative to the horizontal of the pattern drawing. Full size image The principal and secondary directions are presented on the angle histogram plots of Fig. 5e–g . The fibre orientation histograms are in agreement with the force dipole orientation for the three patterns. A sharp peak in the horizontal direction is obtained for [H] pattern, revealing a unidirectional orientation for actin fibres, which corroborates the highly polarized force pattern observed. The angles are spread uniformly in a sector of 90° around the horizontal for [U], showing that fibres can be oriented at different angles from diagonal to horizontal. For [ARROW], the two diagonal directions, especially the one along the adhesive bar (45°) are more probable, but fibres with other directions are also present. In summary, we observed a good correlation between the direction of actin fibres and the traction force orientation. In particular, [H] pattern induced a reproducible orientation of the actin fibres in the horizontal direction. Cell polarization is modulated by contractility We examined the effect of lysophosphatidic acid (LPA) and Y-27632 on actin fibre orientation. LPA is known to activate Rho and stimulates contraction of the acto-myosin cytoskeleton [35] , whereas Y-27632 acts on a Rho-associated kinase (p160ROCK) to inhibit Ca 2+ sensitization and relax cell contractility [36] . After cells are spread on the patterns, LPA (10 μM) or Y-27632 (10 μM) were added and cells were treated for 4 h and 1 h, respectively, before they were fixed and stained for actin. The confocal images obtained on these cells are processed with the method described in the previous paragraph, and the resulting angle histograms are displayed in Fig. 6a . LPA does not seem to significantly change the fibre orientation distribution on the three patterns compared with the control case. In contrast, Y-27632 seems to randomize the angle distributions for [H] and [U] and causes a larger fraction of cells to escape an arrangement with predominantly horizontal fibres. 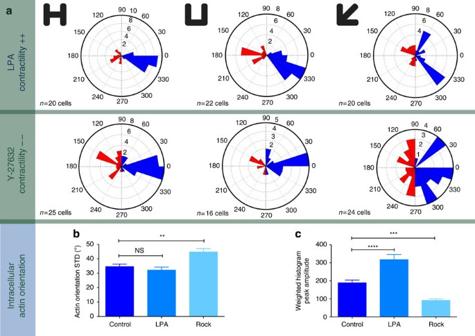Figure 6: Cell contractility modulates actin polarization through RhoA pathway. (a) Histograms showing the principal and secondary actin orientation angle for cells treated with lysophosphatidic acid (LPA) and Y-27632. For the three patterns, while LPA-treated cells retain similar orientation as the one observed in control experiments, Y-27632 treated cells show a broader distribution of actin angles, revealing the role of RhoA in controlling cell polarization. (b) Intracellular orientation fluctuations are quantified by measuring the s.d. of the actin fibre directions on single cell images. LPA slightly reduces this actin orientation fluctuation, while Y-27632 strongly increases intracellular angular variability. (c) Height of peaks in weighted actin angle histograms indicate the degree of orientation of local features in cytoskeletal images. LPA treatment causes actin fibres to be more visible and more clearly oriented, whereas Y-27632 treatment decreases the peaks’ height, indicating that images are locally more isotropic with less visible actin fibres. (Error bars represent s.e.m. *P<0.05, **P<0.01, ***P<0.001 and ****P<0.0001 according to one-way analysis of variance with Tukey’s honestly significant differencepost-hoctest.) Figure 6: Cell contractility modulates actin polarization through RhoA pathway. ( a ) Histograms showing the principal and secondary actin orientation angle for cells treated with lysophosphatidic acid (LPA) and Y-27632. For the three patterns, while LPA-treated cells retain similar orientation as the one observed in control experiments, Y-27632 treated cells show a broader distribution of actin angles, revealing the role of RhoA in controlling cell polarization. ( b ) Intracellular orientation fluctuations are quantified by measuring the s.d. of the actin fibre directions on single cell images. LPA slightly reduces this actin orientation fluctuation, while Y-27632 strongly increases intracellular angular variability. ( c ) Height of peaks in weighted actin angle histograms indicate the degree of orientation of local features in cytoskeletal images. LPA treatment causes actin fibres to be more visible and more clearly oriented, whereas Y-27632 treatment decreases the peaks’ height, indicating that images are locally more isotropic with less visible actin fibres. (Error bars represent s.e.m. * P <0.05, ** P <0.01, *** P <0.001 and **** P <0.0001 according to one-way analysis of variance with Tukey’s honestly significant difference post-hoc test.) Full size image We have also examined intracellular fluctuations of the fibre directions: for each cell, the s.d. of the von Mises distribution used to fit the histogram (width of the peaks as shown in Fig. 5d ) provides an estimation of the variation of fibre orientation. The data for all cells are compared for the three conditions, as shown in Fig. 6b . Treatment by LPA does not significantly reduce the angle fluctuations, but Y-27632 induces a clear increase of intracellular angle fluctuation, meaning that actin fibres have a lower degree of polarization when contractility is inhibited. We believe that the fact that no significant effect is produced by LPA is due to the high degree of cell polarization that is already observed on the patterns, so that further enhancement of contractility by addition of LPA can only produce a small effect. However, LPA does have an effect on stress fibre formation, since, as shown on Fig. 6c , the peaks of the weighted angle histograms obtained for each image is significantly higher after LPA treatment. This means that pixels in the image that form the main peaks have a higher coherency parameter, which denotes a better orientation of the local image features. Therefore, LPA treatment causes actin fibres to be more visible and more clearly oriented, in agreement with previous studies [37] . On the contrary, Y-27632 treatment induces a decrease in the peaks’ height, indicating that images are locally more isotropic with less visible actin fibres, as expected from previous observations [36] . In summary, when acto-myosin contraction is inhibited, fibre orientation in individual cells is more variable and the ability of the patterns to align all cells in one direction is weakened. When cell contractility is stimulated, we observed a slight reduction of intracellular angle fluctuations and a locally more oriented actin organization. Therefore we propose that the modulation of cell contractility through RhoA pathway governs the degree of cell mechanical polarization. We have studied how cells respond to adhesive environments, which differ at the sub-cellular scale while maintaining the same square envelope. To reduce the inherent complexity of living systems, we have deliberately focused on a reductionist system using micro-patterned soft substrates. To uncouple the influence of cell envelope from that of ECM adhesive geometry, we designed patterns that differ on the sub-cellular scale while leading the cells to adopt an envelope of similar shape. Using traction force microscopy, we found that the magnitude and localization of cell-generated forces (the most commonly used output in traction forces studies) are mostly independent of the sub-cellular adhesive environment: the total contractile energy do not change significantly on the different patterns and traction stress are spatially localized in the corners of the square envelope, as expected from the shape of the cell envelope, although stress levels are slightly enhanced at NSF anchors. The influence of ECM adhesive geometry is more clearly revealed by traction force orientation rather than their magnitude. Therefore we have used methods to visualize and quantify force orientation. FOMs make it possible to visualize the stress direction at each location in the cell. To globally assess the polarization of the cell cytoskeleton architecture, the force moment tensor yields the direction of the dominant tractions, as well as the degree of anisotropy of the force pattern. By analyzing both forces and actin fibres orientations, we found a good agreement. These data provide insights into cytoskeleton architecture, in which organization is clearly impacted by sub-cellular ECM geometry: on [H] patterns, most stress fibres are horizontal and connect the two vertical bars, whereas on [U] patterns fibres are oriented in a wide range of directions from horizontal to diagonal, and on [ARROW] patterns fibres are formed along the two diagonal directions and both non-supported edges. Our data suggest that cells are able to sense their adhesive environment and integrate this information at the whole-cell level to organize their internal architecture. Indeed, although [H] and [U] shapes are very similar in the upper part, differences in the actin structure and the local force orientation are observed even in this region, with [H] favouring an unidirectional ordering of the fibres and [U] allowing broadly distributed directions. The polarization of actin cytoskeleton is stimulated by acto-myosin contractility. When examining actin fibre organization, we found larger fluctuations on both intracellular and inter-cellular orientation as the contractility is relaxed. This can be related to previous observations showing that the order parameter of actin cytoskeleton is enhanced when substrate rigidity increases [38] . The observation of a polarized force pattern (unidirectional pinching) on [H] is in contradiction with models [39] , [40] , which predict that traction forces tend to be directed towards the centre of the cell envelope. We demonstrated here that a significant degree of polarization can be induced by the ECM properties. Similar dipolar behaviour with the emergence of a polarized contraction pattern has been experimentally observed in migrating cells, for cells on a rigidity gradient and cells under external anisotropic oscillatory stresses [41] , [42] , [43] , [44] , [45] , [46] , and theoretically modelled [47] , [48] . Here we show that cell polarization can also be induced by the adhesive micro-environment, without changing the cell shape, and that the dipole direction can be precisely controlled. These findings stress the significance of dipolar behaviour in adherent cells [49] . We believe they have important consequences for understanding tissue formation by describing the mechanisms of cell orientation at the single cell level. Our results are also of interest when designing adhesive patterns to control the organization of stress fibres. A number of rules could be derived from this study. For example, the formation of stress fibres seems hindered along adhesive edges: on [U], dominant orientations avoid the vertical bars and prefer directions from diagonal to horizontal; on [ARROW], both vertical and horizontal bars are also avoided, resulting in diagonal directions being favoured. It also seems that, when possible, stress fibres favour an unidirectional order, which ultimately leads to a polarized force pattern: for example, fibres linking diagonal corners are not observed on [H] cells, while they are present on [U] and [ARROW]. Cell culture and labelling MEF cells (kindly provided by O. Destaing and Corinne Albiges-Rizo, Institut Albert Bonniot INSERM U823/ERL CNRS 3148, Grenoble) were cultured in Dulbecco Modified Essential Medium supplemented with 4.5 g l −1 glucose, 2 mM L-glutamine (GIBCO), 10% heat-inactivated foetal calf serum and 0.2% penicillin–streptomycin. Cells were grown in a humidified 5% CO 2 incubator at 37 °C. Cells were seeded on patterned substrates at a density of 5 × 10 4 cm −2 . Micropattern area was adapted to ensure full spreading of MEF cells on each micropattern (900 μm 2 ). Cells not attaching to the adhesive region of the substrate were removed by gentle flushing with fresh media 1 h after seeding. All the traction force measurements or immunostaining were performed 3 h after seeding to ensure a full spreading of the cells. Substrate relaxation was assessed by detaching cells with trypsin. For stress fibre labelling, cells were pre-permealized for 15 s with 0.2% W/V Triton X-100 in cytoskeleton buffer and fixed in 4% paraformaldehyde in cytoskeleton buffer for 10 min to preserve cell shape. Fixed samples were washed three times in PBS. Afterward, cells were stained with fluorescein isothiocyanate-conjugated phalloidin at 1 μM (Sigma-Aldrich). For labelling with primary antibodies, we used rabbit monoclonal anti-paxillin (1:200, anti-rabbit paxillin pTyr 118, Invitrogen 44–722 G). For secondary antibodies, we used fluorescein isothiocyanate-conjugated anti-rabbit (1:200, Jackson ImmunoResearch, West Grove, PA, USA). All steps were performed during 1 h at room temperature in PBS with 3% BSA. Preparations were mounted in Fluoroshield solution (Sigma-Aldrich) to visualize the DNA. PAA micropatterning Micro-patterned PAA hydrogels were fabricated according to a previously described method [28] , detailed hereafter. Round glass coverslips (25 mm) were first cleaned with piranha for 2 h and silanized by dipping in ethanol solution containing 2% (v/v) 3-(Trimethoxysilyl)propyl methacrylate (Sigma) and 1% (v/v) acetic acid for 5 min. After cleaning with ethanol to remove excess silane residue, the coverslips were incubated at 120 °C for 1 h. For Traction Force Microscopy, carboxylate-modified polystyrene fluorescent beads (dark red 200 nm, Invitrogen F-8807) were passivated by poly(ethylene)glycol as follow: fluorescent beads were diluted 25-fold in 2-(N-morpholino) ethane sulfonic acid (MES) buffer (10 mM pH 5.5) containing 8 mg ml −1 N-hydroxysuccinimide (Fluka) and 4 mg ml −1 1-Ethyl-3-[3–dimethylaminopropyl]carbodiimide Hydrochloride (Pierce) before 1:1 mixing with PLL-PEG (PLL(20)-g[3.5]-PEG(2); Susos) solution (4 mg ml −1 in 10 mM pH 8.5 HEPES buffer). The mixture was incubated with rotation at 4 °C overnight. The beads were subsequently spun down and resuspended in HEPES buffer (10 mM pH 7.4). Acrylamide solution containing 6.67% acrylamide and 0.167% bis-acrylamide was mixed with passivated fluorescent beads by sonication before additon of ammonium persulfate (APS) and N,N,N′,N′-tetramethylethylenediamine (TEMED). A drop of acrylamide solution was put directly on the chromium side of the photomask (Toppan). The photomask was cleaned by n-Hexane prior to use to maintain an hydrophobic surface. A silanized coverslip was placed over the drop and let to polymerize for 45 min. The sandwich was then exposed to deep ultraviolet in a UV/Ozone cleaner (Jelight) for 4 min. The coverslip with gel was carefully removed from the mask and incubated with 10 mg ml −1 1-Ethyl-3-[3–dimethylaminopropyl]carbodiimide Hydrochloride and 17 mg ml −1 N-hydroxysuccinimide water solution for 15 min, and then coated with 20 μg ml −1 fibronectin (Sigma) and 5 μg ml −1 Alexa546-conjugated fibrinogen (Invitrogen) in HEPES buffer (10 mM pH 8.5) for 1 h. The photomask was washed with water and then isopropanol. The gel was washed three times by PBS before the seeding of cells. Image acquisition and processing Microscopy experiments were performed using a Nikon Ti-E microscope equipped with an incubator that maintains the temperature at 37 °C, mounted with a CCD camera (Coolsnap, Roper Scientific) and driven with μ Manager. Stained cells were imaged with a Nikon × 63 oil objective lens (numerical aperture 1.4) combined with a 1.5 optical multiplier. To obtain comparable measurements of stress fibres and FAs, cells were plated on a single coverslip containing all micropatterns. The same protocol has been followed for traction force measurements. Image averaging was performed using a home-made Matlab routine. Picture background was subtracted on each picture. After removing the background, the image is binarized. Then only the largest object is kept on the black and white image and black patches inside the cell are filled. The background-subtracted image is normalized by a factor proportional to the integrated intensity in the cell. Finally we chose an averaging level, which is the average intensity level over the whole cell as a fraction of the maximum level. Threshold and average value are kept constant to compare different patterns. For actin orientation quantification, cells have been imaged with a confocal microscope (Leica TCS-SP8) using a × 40 objective (oil immersion, numerical aperture 1.3). Patterned traction cytometry Force calculations on continuous substrates were performed using a method that has been described previously [28] . Briefly, substrate displacements are determined from images of fluorescent beads with and without the adherent cell. After correcting for experimental drift, the images are divided into 6.72 μm square windows. First, cross-correlation is used to yield the average displacement on each pair of subimages, which are shifted accordingly. Then the fluorescent beads are tracked to obtain a displacement field with high spatial resolution. The final displacement field is obtained on a regular grid with 0.84 μm spacing using linear interpolation. Force reconstruction was conducted with the assumption that the substrate is a linear elastic half space, using Fourier Transform Traction Cytometry with zeroth-order regularization [50] . The problem of calculating the stress field from the displacement is solved in Fourier space then inverted back to real space. The final stress field is obtained on a grid with 0.84 μm spacing. All calculations and image processing are performed in Matlab. To calculate and plot mean and s.e. of measured quantities, GraphPad Prism (GraphPad Software, San Diego, CA, USA) was used. Significances were assessed by one-way analysis of variance, using Tukey’s honestly significant difference test to compare every pair of data. How to cite this article : Mandal, K. et al. Cell dipole behaviour revealed by ECM sub-cellular geometry. Nat. Commun. 5:5749 doi: 10.1038/ncomms6749 (2014).